MTSS1is a metastasis driver in a subset of human melanomas In cancers with a highly altered genome, distinct genetic alterations drive subsets rather than the majority of individual tumours. Here we use a sequential search across human tumour samples for transcript outlier data points with associated gene copy number variations that correlate with patient’s survival to identify genes with pro-invasive functionality. Employing loss and gain of function approaches in vitro and in vivo , we show that one such gene, MTSS1 , promotes the ability of melanocytic cells to metastasize and engages actin dynamics via Rho-GTPases and cofilin in this process. Indeed, high MTSS1 expression defines a subgroup of primary melanomas with unfavourable prognosis. These data underscore the biological, clinical and potential therapeutic implications of molecular subsets within genetically complex cancers. The hallmarks of cancer cell biology including metastasis are conferred by genetic or epigenetic modifications of the tumour genome [1] . In some cancers with low mutational complexity, distinct molecular alterations may persist or may be selected for during the course of tumour progression resulting in their high frequency in a given tumour type. The deduced clinical implications can be enormous as documented by the recent therapeutic progress that often relies on attacking the most frequent dominant genetic driver itself or the induced signalling pathway downstream, for example, in chronic myeloid leukemia [2] . On the other hand, clinical, transcriptomic and genetic data [3] , [4] , [5] , [6] have documented an extensive molecular and cellular heterogeneity of several other cancers such as non-small cell lung cancer and melanoma. This molecular diversity may segregate heavily mutagenized cancers [5] , [6] , [7] into different genetic subtypes with distinct cell biology, clinical behaviour and therapeutic response [8] , [9] . In melanoma, several diverse genetic driver alterations, including aberrant gene amplifications as well as mutations, have been identified so far [5] , [6] , [9] , [10] , [11] , [12] . Specific targeting of some of these alterations led to remarkable therapeutic responses [10] , [13] , but is frequently followed by early activation of diverse resistance mechanisms [14] , [15] , [16] , again reflecting the high molecular diversity of this tumour. In addition, a significant proportion of (untreated) melanomas are still left without validated somatic driver alterations. Within heavily mutagenized cancer types, these observations therefore advocate a search for protumorigenic and prometastatic genetic alterations acquired by a subset rather than by the majority of individual tumour samples. Based on frequency and/or uniform distribution of data, conventional frequentist statistics-based approaches are prone to miss genetic alterations that drive tumour subsets. Instead, we subjected tissue-based transcriptomic data to a mathematical algorithm that specifically detects outlier data points and subsequently integrated this information with annotated data on chromosomal copy number gain and patients’ disease outcome. This computational approach was followed by a genetic in vitro screen for cell migration and invasion, assuming that proinvasive genomic alterations are more likely to promote metastasis, the most important prognostic factor for melanoma patients. This integrated gene expression outlier approach identified genes with documented biological function in melanoma and predicted candidate drivers of the disease. An outlier gene satisfying this selection algorithm encoded MTSS1 (MIM, KIAA0429), a regulator of actin and plasma membrane dynamics. Employing gene knockdown and overexpression approaches, we demonstrate here the ability of MTSS1 to promote tumour growth, migration and metastasis of human melanocytic cells. Identification of MTSS1 by an integrated approach The integrated gene expression outlier approach (INDEGO) is inspired by basic principles of the computational copy number and expression algorithm (CONEXIC) [17] that integrates matched copy number and gene expression data from tumour samples to detect biologically relevant gene expression in cancer. INDEGO is based on the following assumptions: (i) in cancers with a highly altered genome, distinct genomic alterations drive subsets rather than the majority of individual tumours; (ii) abnormal (outlier) gene expression signatures could be associated with the presence of genetic driver alterations [17] ; (iii) recurrent non-random copy number alterations can be indicative of the presence of genetic driver alterations [5] , [7] , [12] (iv) driver alterations should have a significant impact on the clinical course of the disease, and (v) the ability to invade the surrounding extracellular matrix allows cancer cells to enter the invasion-metastasis cascade, the most frequent cause of cancer-associated patient mortality [18] .We used INDEGO for a sequential score-guided search across human melanoma samples for transcript outlier data points with associated gene copy number variations that are best correlated with patient’s disease outcome to identify genes that are subsequently screened for functionality in a surrogate assay for cell migration and invasion ( Fig. 1 ). 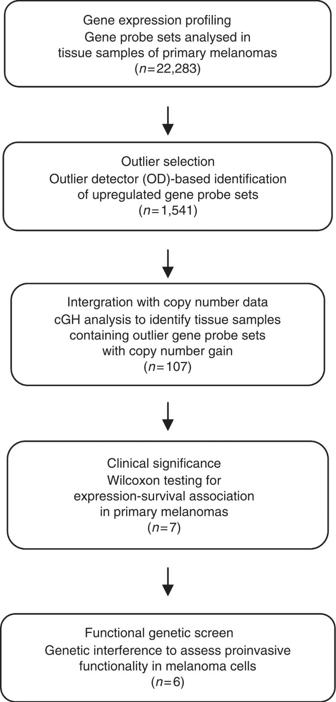Figure 1: The integrated gene expression outlier approach and functional genetic screen for proinvasive activity. Flowchart depicting the multi-tier selection approach for identification of prognosis-relevant proinvasion candidate genes in cancer subsets. Figure 1: The integrated gene expression outlier approach and functional genetic screen for proinvasive activity. Flowchart depicting the multi-tier selection approach for identification of prognosis-relevant proinvasion candidate genes in cancer subsets. Full size image We define an outlier data point as an observation outside the interquartile range of its distribution within a given data set. An outlier detector algorithm (for details see Methods) was used to detect these data points in our previously generated cDNA-microarray expression data set (GEO accession no. GSE8401) from primary human melanoma samples [19] . Here, we focused on data points above the upper quartile of distribution (1,541 outlier probe sets, Fig. 1 ; Supplementary Data 1 ) given the loss-of-function design in the following genetic screening assay. This list of outliers was subsequently intersected with a list of genes residing in recurrent copy number gains (GEO accession no. GSE7606) of the same tissue samples [20] leading to a list of 107 outliers with copy number gain in a subset of melanoma samples ( Fig. 1 ; Supplementary Data 2 ). While genes located in a region of genetic copy gain or loss are indistinguishable in copy number, gene expression patterns permit correlation analyses with a distinct phenotype [17] . To prioritize genes of potential clinical relevance, we used patients’ survival data obtained from annotated clinical data ( Supplementary Table 1 ) and, by Wilcoxon rank-sum testing, found transcripts of 7 ( EIF3H , PDP1 , FZD6 , MTSS1 , LAMP1 , SHC1 and SSR2 ; P <0.05 for each, Table 1 ) of the 107 outliers to be differentially expressed between primary tissues from melanoma patients who subsequently died from the disease and those who did not ( Supplementary Table 1 ). These seven genes were further subjected to a genetic screen in a transwell invasion assay into Matrigel, which simulates extracellular matrix [21] . RNA interference with six ( FDZ6 , MTSS1 , LAMP1 , SHC1 , EIF3H and SSR2 ) of these genes in highly invasive human A375 melanoma cells reduced invasion, with four genes ( MTSS1 , LAMP1 , SHC1 and SSR2 ) showing a reduction by >50% ( Fig. 2a ). Two of these genes have an already proposed or documented role in melanoma cell biology with SHC1 acting on RAS signalling [22] and LAMP1 being implicated in melanoma metastasis [23] , thus supporting the potential biological significance of the applied selection approach. As we were particularly interested in the identification of drivers of the disease and, in contrast to SSR2—an endoplasmic reticulum translocon component [24] , MTSS1’s property (MIM, KIAA0429) to regulate actin and plasma membrane dynamics via interaction with actin [25] , [26] provided a potential link to the phenotype in the invasion assay screen, we decided to study the contribution of MTSS1 to melanoma cell biology in more detail. Table 1 Integrated outlier genes with prognosis-associated expression. 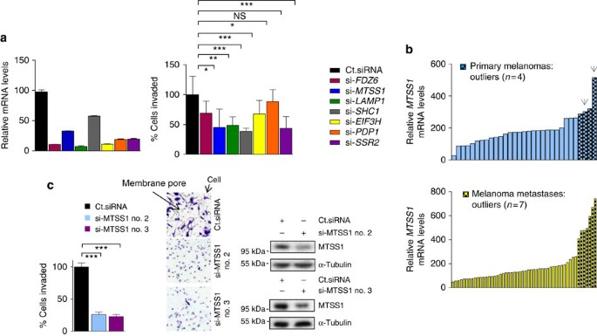Figure 2: Functional screen for proinvasion genes. (a) Left, qRT-PCR to determine mRNA levels of the indicated genes 48 h after RNA interference in human A375 melanoma cells. Relative mRNA levels are shown as percent of control-treated cells (Ct.siRNA). Error bars represent±s.d. calculated from duplicates. Right, invasive potential of human A375 melanoma cells upon RNA interference with expression of the indicated genes as determined in a Matrigel invasion assay. The assay was performed in duplicates. Each bar represents the mean of 12 random microscopic fields±s.d. Data were compared with control-treated cells (Ct.siRNA) using the two-tailed Student’st-test, *P≤0.05, **P≤0.01, ***P≤0.001, NS: not significant. (b)MTSS1transcript levels in human primary and metastatic melanoma samples as obtained from cDNA microarray analysis. Upper panel, primary melanoma (blue,n=31) and lower panel, metastatic melanoma tissue samples (yellow,n=52) plotted along relativeMTSS1transcript levels. Checkered bars represent tissue samples with an outlier expression profile. Arrowheads indicate tissues samples with an underlying copy number gain. (c) Left, invasive potential of human A375 melanoma cells analysed 48 h after RNA interference with control (Ct.siRNA) and additionalMTSS1siRNAs. Bars represent mean±s.d. of three replicates. Relative invasion into Matrigel compared by the two-tailed Student’st-test, ***P≤0.001. Arrows highlight membrane pores and cells. Right, immunoblots show MTSS1 knockdown. Full size table Figure 2: Functional screen for proinvasion genes. ( a ) Left, qRT-PCR to determine mRNA levels of the indicated genes 48 h after RNA interference in human A375 melanoma cells. Relative mRNA levels are shown as percent of control-treated cells ( Ct.siRNA ). Error bars represent±s.d. calculated from duplicates. Right, invasive potential of human A375 melanoma cells upon RNA interference with expression of the indicated genes as determined in a Matrigel invasion assay. The assay was performed in duplicates. Each bar represents the mean of 12 random microscopic fields±s.d. Data were compared with control-treated cells ( Ct.siRNA ) using the two-tailed Student’s t -test, * P ≤0.05, ** P ≤0.01, *** P ≤0.001, NS: not significant. ( b ) MTSS1 transcript levels in human primary and metastatic melanoma samples as obtained from cDNA microarray analysis. Upper panel, primary melanoma (blue, n =31) and lower panel, metastatic melanoma tissue samples (yellow, n =52) plotted along relative MTSS1 transcript levels. Checkered bars represent tissue samples with an outlier expression profile. Arrowheads indicate tissues samples with an underlying copy number gain. ( c ) Left, invasive potential of human A375 melanoma cells analysed 48 h after RNA interference with control ( Ct.siRNA ) and additional MTSS1 siRNAs. Bars represent mean±s.d. of three replicates. Relative invasion into Matrigel compared by the two-tailed Student’s t -test, *** P ≤0.001. Arrows highlight membrane pores and cells. Right, immunoblots show MTSS1 knockdown. Full size image The probe set 203037_s_at corresponding to MTSS1 showed an outlier profile in four out of 31 (13%) primary human melanoma samples ( Fig. 2b , upper panel). From these 31 tumours, array comparative genomic hybridization (cGH) data were available for 25 tumours (80%) comprising three of the four samples with outlier expression. Two of these three samples showed a log2 copy number gain of the corresponding gene locus (8q24.13). When we additionally analysed human melanoma metastases, we observed an outlier profile for this probe set in 7 out of 52 (13%) samples ( Fig. 2b , lower panel), suggesting high expression levels of MTSS1 throughout the metastatic cascade at least in a subset of tumours. In addition, a Cox proportional hazards model analysis showed a statistically significant negative association of MTSS1 transcript levels with survival of primary melanoma patients ( P =0.02; HR=3.734, 95% CI: 1.217–11.455). Finally, in a transwell invasion assay with Matrigel, RNA interference with MTSS1 expression through two additional siRNAs significantly reduced the number of invading human A375 melanoma cells ( Fig. 2c ). Microarray expression data were further confirmed by an additional quantitative real-time (q-RT)-PCR-based analysis of MTSS1 transcript levels in an independent cohort of additional 20 human metastatic melanoma samples ( Supplementary Fig. 1a ) and a panel of 20 different human melanoma cell lines ( Supplementary Fig. 1b ), where we observed a similar differential gene expression profile. Notably, this expression pattern was also portrayed at the protein level in human melanoma cell lines ( Supplementary Fig. 1c ). MTSS1 , melanocytic cell migration, invasion and metastasis We next examined whether MTSS1 enhances the motility of human melanocytic cells by assaying the requirement of MTSS1 for maintaining migration and invasion in cell lines established from human primary melanoma in vitro and the ability of MTSS1 to enhance migration in immortalized human melanocytes in vitro . As expected from the data of the initial genetic screen ( Fig. 2a ), we observed that RNA interference with MTSS1 expression attenuated the ability of human A375 melanoma cells to reconstitute the cell monolayer in an in vitro scratch assay ( Fig. 3a ). Similar results were obtained with human melanoma cell lines WM983A and UACC-257 ( Supplementary Fig. 2 ), which also contain high levels of MTSS1 ( Supplementary Fig. 1c ). We next examined the motility of human melanoma cell line UACC-257 cells by time-lapse video microscopy upon siRNA-mediated interference with MTSS1 expression ( Supplementary Movie 1 ). These cells exhibited oscillating, disoriented movement as compared with control-treated cells, resulting in a reduced net displacement defined as the distance between the starting and the end points of a cell track ( Supplementary Fig. 3 ). 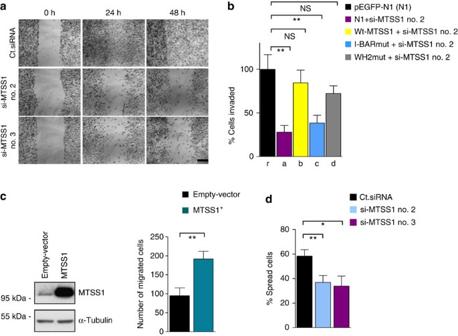Figure 3: MTSS1 promotes melanocytic cell motility. (a)In vitroscratch assay with human A375 melanoma cells 48 h after interference withMTSS1expression by the indicated set of siRNAs. Images were acquired at 0, 24 and 48 h time points after scratching. Scale bar, 350 μm. (b) Representative experiment to rescue the invasive potential of human A375 melanoma cells into Matrigel by expression of wild-type (wt) and mutated (I-BARmut,WH2mut)MTSS1isoforms after RNA interference withMTSS1expression for 48 h. Relative invasion into Matrigel for 20 h as compared with expression of empty-vector (pEGFP-N1) alone by the two-tailed Student’st-test, **P≤0.01, NS: not significant. Bars correspond to mean±s.d. of triplicate data points. (c) Left, immunoblotting for MTSS1 in HMEL cells stably expressing ectopicMTSS1or control empty-vector. Right, migration of empty-vector and ectopicMTSS1-expressing HMEL cells through fibronectin-coated culture inserts for 20 h in the presence of PDGF. The assay was performed in triplicate. Bars represent the mean of five random microscopic fields±s.d. Data were compared using the two-tailed Student’st-test, **P≤0.01. (d) Cell-spreading assay with human A375 melanoma cells for 45 min on fibronectin after 48 h RNA interference withMTSS1expression as determined by the percentage spread of total cells. Bars represent mean±s.d. from three independent experiments. Data were compared with control-treated cells (Ct.siRNA) using the two-tailed Student’st-test, *P≤0.05, **P≤0.01. Figure 3: MTSS1 promotes melanocytic cell motility. ( a ) In vitro scratch assay with human A375 melanoma cells 48 h after interference with MTSS1 expression by the indicated set of siRNAs. Images were acquired at 0, 24 and 48 h time points after scratching. Scale bar, 350 μm. ( b ) Representative experiment to rescue the invasive potential of human A375 melanoma cells into Matrigel by expression of wild-type ( wt ) and mutated ( I-BARmut , WH2mut ) MTSS1 isoforms after RNA interference with MTSS1 expression for 48 h. Relative invasion into Matrigel for 20 h as compared with expression of empty-vector (pEGFP-N1) alone by the two-tailed Student’s t -test, ** P ≤0.01, NS: not significant. Bars correspond to mean±s.d. of triplicate data points. ( c ) Left, immunoblotting for MTSS1 in HMEL cells stably expressing ectopic MTSS1 or control empty-vector. Right, migration of empty-vector and ectopic MTSS1- expressing HMEL cells through fibronectin-coated culture inserts for 20 h in the presence of PDGF. The assay was performed in triplicate. Bars represent the mean of five random microscopic fields±s.d. Data were compared using the two-tailed Student’s t -test, ** P ≤0.01. ( d ) Cell-spreading assay with human A375 melanoma cells for 45 min on fibronectin after 48 h RNA interference with MTSS1 expression as determined by the percentage spread of total cells. Bars represent mean±s.d. from three independent experiments. Data were compared with control-treated cells ( Ct.siRNA ) using the two-tailed Student’s t -test, * P ≤0.05, ** P ≤0.01. Full size image To further analyse the requirement of MTSS1 for directional cell migration and invasion, we again assayed the highly invasive A375 melanoma cells in a transwell invasion assay for their invasive ability through Matrigel. Here, the significantly reduced number of invading cells upon interference with MTSS1 expression could be completely rescued by simultaneous transfection of melanoma cells with a wild-type MTSS1 , but not an empty-vector cDNA ( Fig. 3b ; bars r, a and b). Subsequent gain-of-function assays were performed in HMEL cells (PMEL/hTERT/CDK4(R24C)/p53DD), a TERT-immortalized primary human melanocyte line genetically engineered to ectopically express BRAF V600E and an established cell model to study the contribution of genetic alterations to early stages of melanoma development on a low mutational background [11] , [27] , [28] , [29] . The BRAF V600E background was chosen because of its high frequency in melanoma and any lack of evidence for a preferential association of MTSS1’s copy number gain (cBioPortal for Cancer Genomics; http://www.cbioportal.org/public-portal/index.do ) or functionality ( Supplementary Fig. 4 ) with another, that is, activated NRAS background. HMEL cells expressed low levels of MTSS1 ( Supplementary Fig. 5 ) and, upon stable ectopic expression of MTSS1 , showed a significant increase in the number of migrating cells in a transwell migration assay without induction of cell proliferation ( Fig. 3c and Supplementary Fig. 6 ). As tumour cell migration also requires adhesion to selected extracellular substrates, we also analysed the initial process of cell–matrix interactions, that is, cell spreading [30] . Using fibronectin as a surrogate for extracellular matrix, we performed MTSS1 RNA interference in human A375 and WM983A cells followed by an analysis of their spreading potential [31] . While control cells showed spreading within 45 min after seeding, MTSS1 interference significantly compromised cell spreading at the same time-point ( Fig. 3d and Supplementary Fig. 7 ). Together, these observations demonstrate a promigratory and proinvasive role of MTSS1 in human melanocytic cells in vitro . Promigratory and proinvasive activities are both important prerequisites for tumour progression and metastasis in vivo . Since a gain-of-function (gene overexpression) approach would more closely mimic the clinical scenario, we tested the ability of ectopically expressed MTSS1 to drive distal metastasis in an established cell system to study melanoma metastasis in vivo , namely 1205Lu melanoma cells, a cell line that expresses virtually undetectable levels of MTSS1 ( Fig. 4a and Supplementary Fig. 5 ) and shows weak distal metastasis from skin tumour sites to the lung [28] . As findings at necropsy may fail to detect small and/or anatomically inconspicuous lesions [32] , we used luciferase-based, noninvasive bioluminescence imaging-guided detection of metastasis followed by histological evaluation. To this end, we stably introduced firefly luciferase 2 into ectopic MTSS1- or empty vector-expressing 1205Lu cells ( Fig. 4a ). Cells (1.0 × 10 6 ) were implanted subcutaneously into the flank of athymic nude Foxn1 nu mice. Animals were followed up for 9–10 weeks, a time point at which in our model control tumours developed necrotic cores. At this time, we observed a similar tumour penetrance in both cohorts ( n =9 out of 9 in each cohort, mean tumour volume±s.e.m: 0.71±0.13 × 10 3 mm 3 (empty vector controls) versus 0.70±0.04 × 10 3 mm 3 (ectopic MTSS1 + ), P =0.94, two-tailed Student’s t- test). Animals were examined for metastasis by luciferin-based whole-body in vivo imaging [33] followed by ex vivo imaging of individual organs representing major metastatic sites of melanoma (lymph nodes and distal organ systems such as lung, liver, and so on). Organs suspicious for the presence of metastasis as indicated by imaging were subsequently subjected to whole-organ histological evaluation for metastasis ( Fig. 4b ). Consistent with its promigratory and proinvasive activity in vitro , seven of nine animals (78%) bearing ectopic MTSS1 -expressing melanomas in the subcutaneous sites developed spontaneous micro- and macrometastasis exclusively to the lung, whereas only three of nine animals (33%) in the control cohort harboured metastatic lesions, again exclusively in the lung. 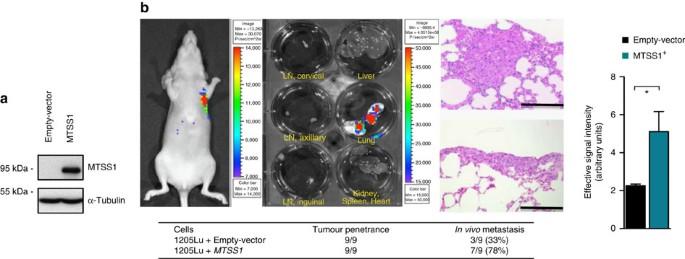Figure 4: MTSS1 promotesin vivometastasis. (a) Immunoblotting for MTSS1 in human 1205Lu melanoma cells stably expressing ectopicMTSS1cDNA or control empty-vector. (b) Left, representative image of luciferase-basedin vivodetection of metastasis from subcutaneous tumours of 1205Lu melanoma cells ectopically expressingMTSS1. The bioluminescence signal is shown here at week 9, the intensity of the signal, measured as photon flux, is shown as a color scale. Middle,ex vivoimaging of individual organs representing known frequent metastatic sites of melanoma. Right, representative H&E lung histology obtained by serial sectioning through the whole organ. Scale bar, 125 μm. Bottom, tumour penetrance andin vivometastasis of empty-vector- and ectopicMTSS1-expressing human 1205Lu melanoma cells. Extreme right, mean metastatic tumour load in animals with empty-vector- versus ectopicMTSS1-expressing cells (measured as photon flux (photons s−1cm−2steradian−1) within the ROI). Error bars represent mean±s.e.m.; *P≤0.05 (two-tailed Student’st-test). Figure 4: MTSS1 promotes in vivo metastasis. ( a ) Immunoblotting for MTSS1 in human 1205Lu melanoma cells stably expressing ectopic MTSS1 cDNA or control empty-vector. ( b ) Left, representative image of luciferase-based in vivo detection of metastasis from subcutaneous tumours of 1205Lu melanoma cells ectopically expressing MTSS1 . The bioluminescence signal is shown here at week 9, the intensity of the signal, measured as photon flux, is shown as a color scale. Middle, ex vivo imaging of individual organs representing known frequent metastatic sites of melanoma. Right, representative H&E lung histology obtained by serial sectioning through the whole organ. Scale bar, 125 μm. Bottom, tumour penetrance and in vivo metastasis of empty-vector- and ectopic MTSS1- expressing human 1205Lu melanoma cells. Extreme right, mean metastatic tumour load in animals with empty-vector- versus ectopic MTSS1- expressing cells (measured as photon flux (photons s −1 cm −2 steradian −1 ) within the ROI). Error bars represent mean±s.e.m. ; * P ≤0.05 (two-tailed Student’s t -test). Full size image Altogether, these in vitro and in vivo complementary gain- and loss-of-function data advocate MTSS1 as a bona fide metastasis driver in human melanoma. MTSS1 and tumour growth As bona fide drivers of melanoma cell migration/invasion and metastasis can also be oncogenic [28] , we next assayed the requirement of MTSS1 for maintaining the tumorigenic phenotype of established human melanoma cell lines in vitro and the ability of MTSS1 to induce tumour growth of immortalized human melanocytes in vivo . When using anchorage-independent in vitro growth as a surrogate for a tumorigenic phenotype, RNA interference with MTSS1 expression in human UACC-257 melanoma cells significantly reduced growth in a 1-week soft agar colony formation assay ( Fig. 5a ). As ectopic MTSS1 doesn’t further increase the a priori high protumorigenic activity of late-stage 1205Lu human melanoma cells (established from lung metastasis) (see Fig. 4b , bottom panel), we utilized HMEL cells to evaluate the tumorigenic capacity of MTSS1 at early stages of melanoma development. Notably, stable ectopic expression of MTSS1 (see Fig. 3c ) significantly promoted the in vivo growth of HMEL xenografts in athymic nude Foxn1 nu mice ( Fig. 5b ). 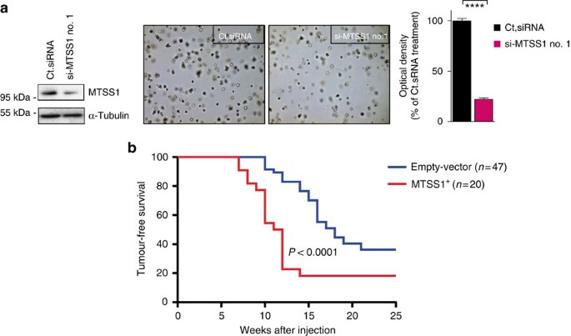Figure 5: MTSS1 exerts protumorigenic activity. (a) Left, immunoblotting for MTSS1 in human UACC-257 melanoma cells after RNA interference withMTSS1expression through the indicated siRNA. Right, short-term soft agar colony formation to assay anchorage-independent growth via AlamarBlue staining. Bars represent mean optical density±s.d. of three replicates. Data were compared using the two-tailed Student’st-test, ****P≤0.0001. (b) Kaplan–Meier tumour-free survival analysis for xenograft assays in athymic nude mice subcutaneously injected with empty-vector- or ectopicMTSS1-expressing HMEL cells in Matrigel. Data were compared using the Log-rank test. Figure 5: MTSS1 exerts protumorigenic activity. ( a ) Left, immunoblotting for MTSS1 in human UACC-257 melanoma cells after RNA interference with MTSS1 expression through the indicated siRNA. Right, short-term soft agar colony formation to assay anchorage-independent growth via AlamarBlue staining. Bars represent mean optical density±s.d. of three replicates. Data were compared using the two-tailed Student’s t -test, **** P ≤0.0001. ( b ) Kaplan–Meier tumour-free survival analysis for xenograft assays in athymic nude mice subcutaneously injected with empty-vector- or ectopic MTSS1- expressing HMEL cells in Matrigel. Data were compared using the Log-rank test. Full size image Altogether, these complementary loss and gain of function data suggest MTSS1 to be required for tumour growth of established human melanoma cells and to be capable of promoting robust tumorigenicity in immortalized human melanocytic cells. MTSS1 -driven cell motility and cofilin activity MTSS1 senses and generates membrane curvature through its N-terminal I-BAR domain (inverse Bin/Amphiphysin/Rvs domain, also known as IRSp53/MIM homology domain or I-BAR/IMD) and interacts with actin monomers through its C-terminal WASP homology 2 (WH2) domain [26] , [34] , [35] . Furthermore, studies by the group of L. M. Machesky demonstrated that MTSS1 mediates activation of Rac via its I-BAR domain [36] , [37] . Rac is a Rho-family GTPase that recruits the Wiskott–Aldrich Syndrome Protein (WASP) family member WAVE to the cell membrane, leading to activation of the Arp2/3 complex and the initiation of actin branching to drive the formation of lamellipodial protrusions and cell motility [38] . Using a transwell invasion assay through Matrigel, we investigated the relative requirement of the MTSS1-I-BAR and the MTSS1-WH2 domains for the invasive ability of human melanoma cells. Based on the previous observation that the reduced invasion of human A375 melanoma cells upon interference with MTSS1 expression could be rescued by transfection with a wild-type MTSS1 cDNA ( Fig. 3b , bars r, a and b), we assayed the contribution of these two domains in reconstitution experiments with corresponding cDNAs carrying loss-of-function mutations [39] . While the actin-binding WH2 mutant showed at least a partial increase of invading melanoma cell numbers, the I-BAR mutant barely rescued cell invasion above levels obtained with an empty vector control ( Fig. 3b , bars c and d). These data support an indispensability of the I-BAR domain for the proinvasive activity of MTSS1 in human melanoma cells. When expressed in melanoma cells, GFP-labelled MTSS1 showed a distinct localization at the cell periphery in addition to the diffuse cytoplasmic distribution previously reported in NIH3T3 cells [35] . A significant fraction of MTSS1 was localized at the front tips of the protruding lamellipodia, but not at the retracting side of the cell, and within filopodial plasma membrane protrusions enriched with Ena/VASP, a protein capping filopodia [40] ( Fig. 6a ), a distribution profile resembling that of actin filament assembly protein cofilin [40] , [41] , [42] . Unphosphorylated active cofilin associates with actin filaments in cell membrane protrusions where it drives actin dynamics by depolymerizing and severing ADP-bound actin filaments to regenerate the pool of actin monomers for new rounds of assembly at filament barbed ends [43] . Furthermore, the severing activity of cofilin is important for generation of the branched actin filament network that drives invasion and metastasis of cancer cells [44] . 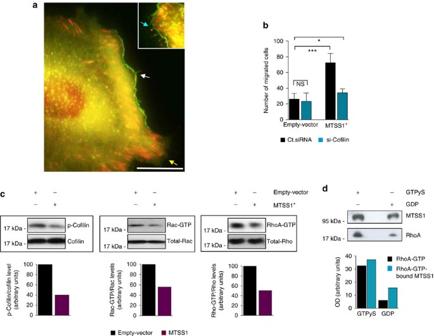Figure 6: MTSS1 interacts with Rho-cofilin signalling pathways. (a) B16 melanoma cell transiently expressing EGFP-MTSS1 (green) together with mCherry-VASP (red). MTSS1 localized in the cytoplasm along with VASP (yellow, overlay of EGFP-MTSS1 and mCherry-VASP), and along the cell periphery of the protruding (white arrow) but not the retracting (yellow arrow) front. Inset, the protruding front of another melanoma cell depicting EGFP-MTSS1 localization in filopodial extensions identified by mCherry-VASP at their tips (cyan arrow). A representative picture is shown from a series of slides. Scale bar, 5 μm. (b) Migration of empty-vector and ectopicMTSS1-expressing HMEL cells through fibronectin-coated culture inserts for 20 h after RNA interference withcofilinexpression for 48 h. Bars represent the mean of five random microscopic fields ±s.d. from three replicates. Data were compared with control-treated cells (Ct.siRNA) using the two-tailed Student’st-test, *P≤0.05, ***P≤0.001, NS: not significant. (c) Left panel, immunoblotting for phospho(Ser3)-cofilin and cofilin levels in empty-vector and ectopicMTSS1-expressing HMEL cells in the presence of fibronectin (10 μg ml−1). Middle panel, pull-down fractions from a Rac activity assay immunoblotted for active (Rac-GTP) and total Rac. Right panel, pull-down fractions from a RhoA activity assay immunoblotted for active (Rho-GTP) and total Rho. Bottom panel, corresponding densitometric plots. (d) Upper panel, pull-down fractions from a Rho activity assay with ectopicMTSS1-expressing HMEL cells in the presence of excess GTPγS or GDP and immunoblotted for MTSS1 and RhoA. Lower panel, densitometric quantification of the immunoblots. Figure 6: MTSS1 interacts with Rho-cofilin signalling pathways. ( a ) B16 melanoma cell transiently expressing EGFP-MTSS1 (green) together with mCherry-VASP (red). MTSS1 localized in the cytoplasm along with VASP (yellow, overlay of EGFP-MTSS1 and mCherry-VASP), and along the cell periphery of the protruding (white arrow) but not the retracting (yellow arrow) front. Inset, the protruding front of another melanoma cell depicting EGFP-MTSS1 localization in filopodial extensions identified by mCherry-VASP at their tips (cyan arrow). A representative picture is shown from a series of slides. Scale bar, 5 μm. ( b ) Migration of empty-vector and ectopic MTSS1- expressing HMEL cells through fibronectin-coated culture inserts for 20 h after RNA interference with cofilin expression for 48 h. Bars represent the mean of five random microscopic fields ±s.d. from three replicates. Data were compared with control-treated cells ( Ct.siRNA ) using the two-tailed Student’s t -test, * P ≤0.05, *** P ≤0.001, NS: not significant. ( c ) Left panel, immunoblotting for phospho(Ser3)-cofilin and cofilin levels in empty-vector and ectopic MTSS1- expressing HMEL cells in the presence of fibronectin (10 μg ml −1 ). Middle panel, pull-down fractions from a Rac activity assay immunoblotted for active (Rac-GTP) and total Rac. Right panel, pull-down fractions from a RhoA activity assay immunoblotted for active (Rho-GTP) and total Rho. Bottom panel, corresponding densitometric plots. ( d ) Upper panel, pull-down fractions from a Rho activity assay with ectopic MTSS1- expressing HMEL cells in the presence of excess GTPγS or GDP and immunoblotted for MTSS1 and RhoA. Lower panel, densitometric quantification of the immunoblots. Full size image To establish a causal relationship between cofilin activity and MTSS1-driven migration of human melanocytic cells, we first assayed whether cofilin silencing would abolish the enhanced migration observed in HMEL cells ectopically expressing MTSS1 . While siRNA-mediated interference with cofilin expression in empty vector control HMEL cells did not affect the number of migrated cells, HMEL cells stably expressing MTSS1 showed reduction of migrated cells almost to the level observed in control cells ( Fig. 6b ). Consistently, ectopic expression of MTSS1 in HMEL cells reduced the cellular levels of phospho(Ser3)-cofilin ( Fig. 6c , left panel), a phenomenon also observed in human Lu1205 melanoma cells ( Supplementary Fig. 8a ). Conversely, siRNA-mediated interference with MTSS1 expression induced phospho(Ser3)-cofilin levels in HMEL as well as in human A375 melanoma cells ( Supplementary Fig. 8b ), thus complementing our observations from gain-of-function assays. The known ability of active Rac to phosphorylate cofilin through a sequential activation of p21-activated protein kinase (PAK) and LIM domain kinase (LIMK) [45] and the observed indispensability of the Rac-interacting I-BAR domain for MTSS1’s pro-invasive ability ( Fig. 3b ) pointed towards a MTSS1–Rac–Cofilin wiring. We therefore investigated a possible modulation of Rac activity through MTSS1. While ectopic expression of MTSS1 in HMEL cells markedly subdued the levels of p(Ser3)-cofilin ( Fig. 6c , left panel), GTP-bound Rac levels showed only a subtle drop ( Fig. 6c , middle panel). Even though this observation does not categorically exclude a functional coherence between Rac activity and phospho-cofilin levels, it prompted us to study the contribution of other established signalling pathways. In addition to the Rac–PAK–LIMK axis, the RhoA-Rho-associated protein kinase (ROCK)-LIMK signalling cascade regulates cofilin phosphorylation and activation to diminish cell migration [43] , [46] . First, suppression of inactive phospho(Ser3)-cofilin levels upon pharmacological inhibition of ROCK confirmed an intact RhoA-ROCK-LIMK-cofilin signalling in human A375 melanoma cells ( Supplementary Fig. 8c ). More importantly, upon ectopic expression of MTSS1 , HMEL cells exhibited lower levels of active GTP-bound Rho ( Fig. 6c , right panel), correlating well with the reduced cellular levels of phosphorylated cofilin. To garner a further mechanistic understanding of the interplay between RhoA and MTSS1, we investigated a potential interaction between the two proteins in HMEL cells stably expressing ectopic MTSS1 and observed in a pulldown for active-RhoA, a co-precipitation of MTSS1 at levels commensurate to that of active-RhoA ( Fig. 6d ). These results speak for an engagement between RhoA and MTSS1 in human melanocytic cells and further substantiate the functional role of MTSS1 in melanocytic cell motility. Metastatic melanoma is a highly aggressive disease with an eventually fatal outcome. Considering the extensive molecular and cellular heterogeneity of this tumour, we applied in this study a sequential explorative approach specifically designed to identify biologically and clinically relevant genetic alterations that drive subsets rather than the majority of tumour samples within a given cancer type. The identification of genes with documented impact on melanoma biology along with potentially proinvasive drivers of the disease demonstrates the strength of the chosen approach as well as its complementarity to previous searches within the majority of tumour sample sets [28] . MTSS1 combines protumorigenic and proinvasive activities in melanocytic cells and thus seems to belong to the recently described group of oncogenic metastasis drivers in melanoma [28] . Consistent with the hypothesis that this kind of biological information can inherently be carried already in the genome of early-stage melanomas [28] , [47] , [48] , we observed an outlier expression pattern of MTSS1 to coincide with the presence of a copy number alteration at 8q24.13 in a subgroup of primary melanoma samples. The 8q24.13 gene locus seems to carry a certain degree of susceptibility to genetic alterations as it has been identified as a papillomavirus integration site in cervical carcinoma [49] , a translocation site in patients with genetic disorders such as the 22q11.21 deletion syndrome [50] and a site of copy number gain in cancers of prostate [51] , gastroesophageal junction [52] and breast [53] . Initial expression–phenotype association studies showed a downregulated or lost expression of MTSS1 in cancer cells of bladder [54] , [55] and prostate [56] . These data were subsequently challenged by several other studies that showed a rather preserved and at times even increased expression of MTSS1 in human tumour cell lines from bladder, breast and prostate [37] as well as individual tissue samples from cancers of head and neck [36] , esophagus [57] , breast [58] , liver [59] and medulloblastomas [60] . These observations could be suggestive for the presence of a similar (MTSS1-driven) molecular subtype in cancers other than melanoma, a hypothesis further strongly supported by large-scale, integrated cancer genomic data sets that describe MTSS1 copy number gain in at least a subgroup of tumour samples from almost all analysed cancer types (in 34 of 38 studies (cBioPortal for Cancer Genomics; http://www.cbioportal.org/public-portal/index.do , as of Oct 2013). While biochemical data provide a profound basis for a proinvasive activity of MTSS1 (refs 25 , 26 , 37 ), there are contrasting observations regarding the protumorigenic and promigratory functionality of MTSS1 in individual cancer sublines within [58] and between individual reports [36] , [37] , [58] . So far, however, rigorous evaluations of MTSS1’s requirement for in vivo migration and metastasis of cancer cells have been lacking. Together with our data, these observations encourage a more detailed functional evaluation of MTSS1 in individual cancer cell contexts and underscore the potential value of the integrated gene expression outlier approach for the identification of further molecular subsets in melanoma and other cancer types. In addition to its direct interaction and reorganization of the actin cytoskeleton through its I-BAR domain, another promigratory mechanism has most recently been ascribed to MTSS1 in Drosophila , namely orchestration of directional migration through impairment of endocytosis of ligands for receptor tyrosine kinases EGF- and PDGF/VEGF-like-receptors [61] . There, live-imaging experiments revealed that an absence of MTSS1 is associated with impaired directional migration in response to EGF and PDGF. We share this latter observation in loss-of-function experiments and further support it by gain-of-function experiments in human melanocytic cells proposing MTSS1 -driven directional migration as a cross-species conserved mechanism. Both Rac-PAK-LIMK and RhoA-ROCK-LIMK signalling tracts have been shown to regulate cofilin activity [45] , [46] and our results propose MTSS1 -associated regulation of cofilin activity to utilize both of these signalling modules. Physical interaction between MTSS1 and Rac has been documented earlier; to the best of our knowledge, however, RhoA-MTSS1 engagement has previously not been reported. While these data are supported by observations from other cell lines where ectopic expression of MTSS1 or its I-BAR domain results in reduction of stress fibers [35] , a hallmark phenotype for RhoA inactivation [62] , they do not exclude additional indirect Rac and RhoA regulation through MTSS1 by affecting the geometry or lipid distribution of the leading edge plasma membrane through its I-BAR domain [26] or by altering the structure of the actin cytoskeleton through its interactions with cortactin or Daam1 formin [63] , [64] . It is also interesting to note that in contrast to earlier reports about MTSS1 to activate Rac [37] , but consistent with Rac’s dispensability for I-BAR-induced filopodia formation [34] , we observed a reduction of Rac activity in HMEL cells upon MTSS1 expression. In addition to the use of different cell systems, the contextual role of extracellular cues such as fibronectin as used in our study could be a critical determinant of modulation of Rac activity by MTSS1. The latter observations demand caution to extrapolating a similar functionality of MTSS1 across diverse cancer types. In addition to overexpression, the interplay of MTSS1 with other components of the cytoskeletal machinery to confer cell mobility is subject to a high degree of regulation. This includes (i) the extent of alternative splicing leading to the expression of MTSS1-isoforms composed of different functional domains [60] , (ii) the degree of expression of, substitution by and/or competition with other BAR domain protein family members and lipid-binding proteins [65] that interfere with binding of MTSS1 to its substrates such as Cortactin [61] , [63] , (iii) the level of competition with other actin-binding adaptor molecules such as N-WASP for binding to active actin monomers [63] and (iv) presumably the expression of MTSS1’s substrates in different cellular contexts. In conclusion, we report a molecular subtype of human melanoma and, consistent with the concept of oncogenic metastasis drivers in early-stage melanoma [28] , demonstrate a protumorigenic, promigratory and prometastatic role of MTSS1 in human melanocytic cells. The presence of this genetic alteration already in primary melanoma tissues could allow early detection of patients with an unfavourable prognosis presumably due to an increased risk of metastasis. Our data further advocate interference with both Rac-PAK-LIMK and RhoA-ROCK-LIMK signalling as one mode of action of MTSS1, which may help to guide the development of an early, precise and pathology-adjusted therapeutic intervention. Plasmids The constructs for retroviral transduction were cloned using the Gateway system (Invitrogen). For generating the gateway entry clone the MTSS1 sequence was amplified from a plasmid DNA construct harbouring murine MTSS1 cDNA (Gene Bank NM_144800), using the following primers, forward: 5′-Ggggacaagtttgtacaaaaaagcaggctccgaggctgtgatcgagaagg- 3′ and reverse: 5′ -Ggggaccactttgtacaagaaagctgggtctaagagaagcgcggtgc- 3′. The forward primer was designed to enable N-terminal Strep HA-Tag fusion when using the destination vector pfMIG-gw (kindly provided by F. Grebien, Center for Molecular Medicine, Austrian Academy of Sciences, Austria). Enhanced green fluorescent protein (EGFP) fusions of wild-type mouse MTSS1 were generated by cloning the MTSS1 cDNA into the pEGFP-C3 vector (Clontech) using the BsrGI restriction site. MTSS1 mutants, IMDmut (K146A, K149A, K150A) and WH2mut (K746A, K747A), have been generated previously [34] , [35] . Transient transfections into human melanoma cells were performed using Lipofectamine (Invitrogen) according to the manufacturer’s instructions. Antibodies The following antibodies were used: human MTSS1 (2G9) (dilution, 1:1,000) from Abnova; MTSS1 (P549) (dilution, 1:1,000), phospho(S3)-cofilin (dilution, 1:1,000), cofilin (clone D3F9) (dilution, 1:1,000) from Cell Signaling Technology; Rac1 (Clone 102) (dilution, 1:1,000) from BD Pharmingen, Rho (1:1,000) from Thermo Scientific and α-Tubulin (DM1A) (dilution, 1:1,000) from Calbiochem. RNA extraction and quantitative real-time PCR Total cellular RNA was extracted using TRI Reagent (Sigma-Aldrich) according to the manufacturer’s protocol, and 1 μg per sample was subjected to reverse transcription, using Superscript II Reverse Transcriptase (Invitrogen). TaqMan gene expression assays for MTSS1 and Ubiquitin C were ordered from Applied Biosystems ( MTSS1 : Hs00207341_m1, Hs01036424_m1, UBC : Hs00824723_m1, EIF3H : Hs00186779_m1, PDP1 : Hs01081518_s1, SSR2 : Hs00162346_m1, Actin : Hs99999903_m1). A StepOne Plus qT-PCR System was used for amplification (2 min 50 °C; 10 min 95 °C; 40 cycles: 15 s 95 °C, 1 min 60 °C) and detection. Reverse transcription negative controls were always included. For relative quantification of gene expression, the 2− ΔΔCT method was used. Analysis of transcript profiles Microarray probe intensity data were previously generated from 83 fresh primary and metastatic human melanoma tissue samples [19] . Data are accessible through GEO Series accession no. GSE8401. Data were read from Affymetrix CEL files and processed with the Genespring GX11.5 software (Agilent Technologies Inc.). To obtain a reasonable number of data points for individual transcripts, only probe sets showing ≥80% p-calls in the primary tumour sample set ( n =6,904) were used for further calculation. The outlier detector algorithm defines an outlier as any observation outside the range: ( Q 1 −k ( Q 3 −Q 1 ), Q 3 +k ( Q 3 −Q 1 )) for constant k =1 with Q 1 and Q 3 as the lower and upper quartiles, respectively. A tumour subset was confined to at least 7.5% and not more than 20% (3–6 out of 31) tissue samples. Consequently, we specified candidate outlier probe sets by expression signals outside the previously defined range present in at least 7.5% and not more than 20% tissue samples. As we used a loss-of-function design in the following screening assay, we selected outliers above the upper quartile of distribution. Array cGH data analysis Array cGH profiles of most transcript-profiled human tissue samples (25 out of 31, 80%) are part of a reported series of 101 fresh primary and metastatic human melanoma, melanocytic nevi and normal skin tissue samples [20] and are available online at GEO under super-series accession no. GSE7606. Microarray and cGH probe set IDs were mapped with the db2db-tool ( http://biodbnet.abcc.ncifcrf.gov/db/db2db.php ). We set up a list of candidate outliers for each individual tumour sample and intersected this list with a list of genes residing in recurrent copy number gains as defined by a log2 ratio ≥0.4 signal amplification event [20] from the same tissue sample. Candidate outliers qualified as integrated outliers only, if present in the intersection of at least one tissue sample (that is, at least 16% of samples within a potential tumour subset, for definition of a tumour subset see above). Given the previous selection for upregulated outliers (see above), we focused on copy number gains in this analysis. Patient groups comparison and survival times analysis Transcriptomic data were annotated with clinical information including a follow-up ranging from 5–147 months ( Supplementary Table 1 ). For these studies already published cGH, gene expression and clinical data were utilized [19] , [20] . The corresponding samples were collected from 1992 to 2001 as a part of the diagnostic workup or therapeutic strategy. The research was approved by the institutional review board at the University of Essen and granted an exemption. Informed written patient consent was obtained for all tissues in accordance with the ethical standards laid down in the 1964 Declaration of Helsinki. Comparison of patients groups for transcript levels was done individually with each integrated outlier by Wilcoxon testing. Since we analysed upregulated outliers, one-sided testing was performed with a significance level set to P <0.05. Integrated outliers were subsequently ranked as to P values to prioritize for further experimental validation. To evaluate the association of expression levels with survival times of primary melanoma patients, the Cox proportional hazards model [66] with the pre-specified endpoint (death from disease), the time from first diagnosis to documented death and censored time values (time from first diagnosis to last clinical visit) for surviving patients were used. The PHREG procedure of the SAS System V9.2 (SAS Institute Inc.) was used for statistical computations and the significance level for model results was set to P <0.05. Cell culture and genetically modified cell lines All cell lines were maintained in RPMI containing 10% fetal calf serum (FCS). Ectopic MTSS1 -expressing- and empty vector-HMEL cells are immortalized human PMEL/hTERT/CDK4(R24C)/p53DD/BRAF (V600E) melanocytes [11] genetically modified to ectopically express MTSS1 or the corresponding empty vector alone. Ectopic MTSS1-expressing or empty vector 1205Lu cells are human 1205Lu melanoma cells (obtained from the American Type Culture Collection) genetically modified to ectopically express MTSS1 or the corresponding empty vector alone. For retrovirus production, 293-GP cells were transfected with 6 μg of the N-Strep-HA-MTSS1-IRES-GFP/pfMIG-gw construct (for plasmids, see below) together with 1 μg of pVSV-G using Polyfect transfection reagent (Qiagen) according to the manufacturer’s instructions. After 12–16 h, the supernatant was replaced by fresh medium and virus production allowed for 24 h. Virus containing supernatant was filtered and used directly for the transduction of human cells. After three passages, cell lines were tested for green fluorescent protein (GFP) and transgene expression using flow cytometric analysis and western blotting. An almost pure population (>98%) of transduced cells was obtained by FACS-based sorting of GFP-positive cells. siRNA transfections Small interfering RNAs (siRNAs) targeting human MTSS1 s18916 (no. 1), 21918 (no. 2), 138403 (no. 3), FDZ6 (s729), SHC1 (s21811), LAMP1 (s8082), EIF3H (s16507), PDP1 (s29328), SSR2 (s13481), cofilin (s2937) and respective control nontarget siRNA no. 2 (Ct.) and Silencer Negative Control no. 1 siRNAs were purchased from Ambion (Applied Biosystems). Please see Supplementary Table 2 for the corresponding siRNA sequences. Transient siRNA transfection was performed using Lipofectamine 2000 (Invitrogen) according to the manufacturer’s instruction. Western blotting and pulldown assays Total protein was extracted in Laemmli buffer, fractionated by SDS polyacrylamide gels and transferred to Immobilon-P PVDF membranes (Millipore) by semidry electro-transblotting (Hoefer Scientific). After blocking with 5% non-fat dry milk (Bio-Rad), the membranes were incubated with primary antibodies, overnight at 4 °C. Depending on the primary antibody used membranes were incubated with HRP-conjugated goat-anti-mouse or goat-anti rabbit antibody (1:40,000; BioRad) for 1 h at 20 °C. Membranes were incubated with HRP-conjugated goat-anti-mouse antibody (1:40,000; BioRad) for 1 h at 20 °C. Protein signal was visualized using the ECL detection system (Pierce) according to the manufacturer’s instructions. The full blots corresponding to the most important western blots are shown in Supplementary Fig. 9 . Pulldown of active Rho was performed using Active Rho Pull-Down and Detection Kit (Thermo Scientific) according to the manufacturer’s instructions. Briefly, cells were lysed for 5 min on ice using 25 mM Tris–Cl, pH 7.2, 150 mM NaCl, 5 mM MgCl 2 , 1% NP-40 and 5% glycerol followed by centrifugation at 16,000 g at 4 °C for 15 min. GST-Rhodekin-RBD was bound to Glutathione Resin and incubated with 500 μg protein lysate for 1 h at 4 °C with gentle rocking followed by three washing steps to remove unbound proteins. Captured proteins were solubilized in SDS sample buffer and heated to 95 °C for 5 min before electrophoresis. For GTPγS or GDP treatment lysates were incubated with GTPγS at a final concentration of 0.1 mM or GDP at a final concentration of 1 mM at 30 °C for 15 min with agitation. To terminate the reaction the samples were placed on ice and MgCl 2 to a final concentration of 60 mM was added. Fluorescence microscopy Melanoma cells were transiently transfected with EGFP-wtMTSS1 cDNA together with mCherry-VASP cDNA construct. Cells were grown overnight and plated on fibronectin-coated glass coverslips. For image acquisition, an Axiovert 200M inverted microscope (Zeiss) was used, equipped with a rear-illuminated CCD camera (Roper, 16 μm px −1 ) controlled by MetaMorph 7.5 software (Molecular Devices). Anchorage-independent growth Soft agar colony formation was assessed in triplicates in a fluorescence-based 1-week assay. Briefly, 96-well plates coated with bottom agarose prepared with 0.5% agarose in RPMI plus 10% FCS. Twenty-four hours after transfection with siRNA, 2 × 10 3 cells per well were added in top agar prepared with 0.4% agarose in RPMI plus 10% FCS and subsequently covered with RPMI plus 10% FCS and penicillin/streptomycin (Invitrogen). After 7-day incubation, colonies were stained with AlamarBlue (Invitrogen) according to the manufacturer’s instructions and fluorescence read with excitation at 530 nm and emission at 590 nm using a multiwell plate reader. In vitro scratch assay siRNA-transfected melanoma cells were allowed to grow to confluence (usually 48 h post transfection). Subsequently, a pipette tip was used to scratch the cell monolayer. The cell monolayer was washed and re-fed with fresh medium plus 10% FCS and thymidine (Sigma-Aldrich). Immediately following scratching (0 h) and after incubation of cells at 37 °C for 24, 36 and 48 h, phase-contrast images ( × 10 field) of the scratch were photographed digitally with an Olympus BH-2 inverted phase contrast microscope ( × 4 objective), equipped with an E-330 digital camera (Olympus). Invasion and transwell migration assays Invasion assays were performed 48 h after siRNA transfections using BioCoat Matrigel Invasion Chambers with 24-well plate format and 8-μm pore size (BD Biosciences), as per manufacturer’s instructions. Control inserts without Matrigel were used to account for seeding differences. Cells were added to the upper chamber in serum-free DMEM with thymidine (2 × 10 4 cells in 500 μl). The lower chamber contained DMEM containing 10% FCS. Following an incubation for 20 h at 37 °C at 5% CO 2 , membranes were fixed and stained using the Kwik-Diff Staining kit (Thermo Fisher Scientific) according to the manufacturer’s instructions followed by counting of cells at the bottom surface. In each experiment, 9–12 randomly selected fields at a × 10 or × 20 magnification were counted. For transwell migration assays, cells were serum-starved overnight. Following trypsin treatment, washing in RPMI and incubation at 37 °C for 30–60 min, 4 × 10 3 cells in 500 μl RPMI were plated per 8-μm pore-sized cell culture insert (BD Biosciences) coated with 10 μg ml −1 FN. The lower chamber contained 750 μl RPMI plus 20 ng ml −1 PDGF. Incubation and cell counting were performed as described for the invasion assay. Cell spreading assay Forty-eight hours post siRNA treatment, cells were allowed to spread at 37 °C for 45 min [31] . Cells attached to coverslips were stained with Alexa Fluor 488 phalloidin (Molecular Probes, Invitrogen) and visualized using an Axiovert 200M microscope (Zeiss) [67] . Unspread cells were defined as round phase-bright cells, whereas spread cells were defined as elongated or flattened phase-dull cells with extended membrane protrusions and a total diameter more than twice the diameter of the nucleus. In each experiment, at least 3 × 15 cells were counted. Time-lapse imaging Briefly, UACC-257 melanoma cells were transfected with Ct. or MTSS1 siRNA no. 3. Additional controls included untreated as well as Lipofectamine-treated UACC-257 cells. Twenty-four hours post transfection, cells were seeded at a density of 3 × 10 4 –2.4 × 10 5 cells per cm 2 in 24-well plates and cultured in RPMI plus 10% FCS for 24 h. Thereafter, the cluster plates were transferred to a heated (37 °C), gassed (5% CO 2 ) and humidified chamber fitted onto an inverted microscope (Leica DM IRE2 HC Fluo) with a motorized cross-stage (Maerzhaeuser). Images of each well were recorded every 10 min over the next 36 h using a × 10 objective ( × 10/0.22 LMC−/−7.8 100 objective, Leica) with a digital camera (Leica DFC350FX). Recordings were stored with the FW4000 database software (Leica). All image processing was performed using ImageJ software (NIH; http://rsb. 106 info.nih.gov/ij/ ) [68] . For recording and analysing the cell path, ImageJ plug-in MTrackJ was used ( http://www.imagescience.org/meijering/software/mtrackj/ ). Each kind of treatment and cell density was followed in three independent time-lapse movies. ( 3 H)-Thymidine incorporation A total of 2,000 cells per well were plated in the 96-well format and cultured for 6 days. On day 6 3H-Thymidine (New England Nuclear) was added at a final concentration of 2 μCi ml −1 . After 20 h incubation the cells were harvested using Tomtec harvester (HVD Life Sciences) and counted using a beta-scintillation counter (HVD Life Sciences). In vivo tumour assays All experiments were performed in female, 6–8 weeks, athymic nude Foxn1 nu mice (Harlan-Winkelmann) with the approval and following the guidelines of the Animal Research Committee of the Medical University of Vienna and the Austrian Ministry of Science and Research. For xenograft tumorigenicity studies, 3.0 × 10 6 cells (in 200 μl of 7 mg ml −1 Matrigel, BD #354234) were injected subcutaneously into the flanks of mice and tumour growth monitored on a regular basis. For in vivo imaging of xenograft metastasis studies, we first generated ectopic MTSS1- and control empty vector 1205Lu melanoma cells stably expressing firefly luciferase 2 (FLuc2). The vector pLB-U-FLuc2 was generated by Invitrogen Gateway cloning reaction of pE-FLuc2 (entry vector) and pLB-U-DEST (destination vector) according to the manufacturer’s protocol (Gateway Clonase II Enzyme Mix, Invitrogen). The entry vector pE-FLuc2 was created by replacing eGFP of pE-eGFP with the NcoI and XbaI FLuc2 fragment of pGL4.10-Basic (Promega). pE-eGFP was generated by cloning the eGFP fragment from pFUGW into pENTR-A1 via BamHI and EcoRI sites. To create pLB-U-DEST, several subcloning vectors were generated. pFUBW was created by cloning a PCR product of the blasticidin cassette of pLentiDest6 (Invitrogen) into pFUGW, replacing eGFP using BamHI and EcoRI sites. Subsequently, the gateway cassette from pGW2for was excised with NheI and XbaI and cloned upstream of the blasticidin cassette of pFUBW into the NheI site to created pLB-U-DEST. pGW2for was created by cloning a PCR product of the gateway cassette into pBluescript(II)-KS(+) (Stratagene). pLB-U-FLuc2 was introduced into melanoma cells by retroviral transduction and transduced cells selected against blasticidin. Luciferase activity was confirmed in vitro with the Xenogen IVIS 50 imaging system (Caliper Life Sciences) by the addition of 0.03 mg of D -Luciferin to serially diluted cell numbers. Ectopic MTSS1- and empty vector 1205Lu melanoma cells showed equal cell proliferation before xenografting. For in vivo imaging, briefly, 1.0 × 10 6 cells were implanted subcutaneously into the flank of mice and bioluminescent imaging was performed once a week 10 min after i.p. injection of 100 μl D -Luciferin (15 mg ml −1 in PBS) using the Xenogen IVIS 50 in vivo imaging system [33] . Animals were anaesthetized by intraperitoneal injection of ketamine (80 mg per kg) and xylazine (10 mg per kg) and were placed in the supine position. At the end of the experiment, imaging was performed by injection of 200 μl of D -Luciferin and removal of the primary tumour to minimize metastasis-unrelated signals. Binning was set to high sensitivity (HS(8)), field of view to 15 × 15 cm and exposure time to 5 min. Thereafter, organs were excised from each mouse and individually subjected to ex vivo imaging. Analysis was performed using LivingImage software (Caliper) by measurement of photon flux (measured in photons s −1 cm −2 steradian −1 ) with a region of interest (ROI) drawn around bioluminescence signals. For lung metastasis, an ROI was used encompassing the thorax of the mouse. For determination of the ‘fold increase’ above background, average background measurements were obtained using the same ROI on a corresponding region from control mice. For histological confirmation of detected bioluminescence signals, individual organs were collected immediately after ex vivo imaging in formalin and embedded in paraffin. Serial sections of 5 μm in thickness were taken every 50 μm through the whole organ and stained with hematoxilin & eosin (Merck). Statistical methods Statistical significance between two groups was assessed by the two-tailed Student’s t- test. GraphPad Prism 5 software (Graphpad) was used for to perform all statistical calculations as well as to generate Kaplan–Meier curves for in vivo experiments and to calculate the respective Log-rank testing. How to cite this article: Mertz, K. D. et al. MTSS1 is a metastasis driver in a subset of human melanomas. Nat. Commun. 5:3465 doi: 10.1038/ncomms4465 (2014).